An orbital-selective spin liquid in a frustrated heavy fermion spinel LiV2O4 The pronounced enhancement of the effective mass is the primary phenomenon associated with strongly correlated electrons. In the presence of local moments, the large effective mass is thought to arise from Kondo coupling, the interaction between itinerant and localized electrons. However, in d electron systems, the origin is not clear because of the competing Hund's rule coupling. Here we experimentally address the microscopic origin for the heaviest d fermion in a vanadium spinel LiV 2 O 4 having geometrical frustration. Utilizing orbital-selective 51 V NMR, we elucidate the orbital-dependent local moment that exhibits no long-range magnetic order despite persistent antiferromagnetic correlations. A frustrated spin liquid, Hund-coupled to itinerant electrons, has a crucial role in forming heavy fermions with large residual entropy. Our method is important for the microscopic observation of the orbital-selective localization in a wide range of materials including iron pnictides, cobaltates, manganites and ruthnates. Electrons in metals behave as quasiparticle, whose mass often becomes extremely heavy when metallic phases are close to the quantum critical boundary for the insulating or magnetic phase [1] . The microscopic understanding of heavy quasiparticles (HQs) has been a goal of modern many-body quantum statistics. An established route for HQs is antiferromagnetic Kondo coupling between localized f spins and itinerant electrons in rare earth metals. In contrast to the f -electron case, the presence of localized spins is not apparent for d -electron systems. Alternative routes driving d HQ formation have been challenging issues in strongly correlated electron physics. A representative d HQ material is the vanadium spinel LiV 2 O 4 (refs 2 , 3 ), which has a highly frustrated pyrochlore lattice for the B site V 3.5+ (3 d 1.5 ) ions ( Fig. 1a ). Anisotropic orbital-dependent intersite interactions give an itinerant orbital and a more localized a 1g orbital through a small trigonal distortion of the VO 6 octahedron ( Fig. 1b ) [4] , [5] . The HQ was initially explained by off-site Kondo exchange interactions, J K , between localized a 1g moments and itinerant electrons ( Fig. 1b ) [4] . In the t 2g manifold, however, the strong on-site ferromagnetic Hund's exchange interaction, J H , can overcome J K . Many alternative scenarios, such as geometrical frustration via antiferromagnetic interactions J AF , [6] , [7] , [8] , electron correlations [9] , [10] and spin-orbital fluctuations [11] , [12] have been proposed. 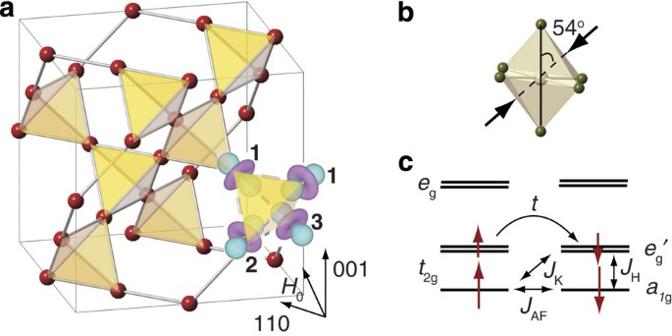Figure 1: V pyrochlore lattice and exchange interactions between 3dorbitals in LiV2O4. (a) Corner-sharing V tetrahedra offer geometric frustration against magnetic ordering. In the cubic lattice with local trigonal distortion, three vanadium sites witha1g-like orbitals, numbered1,2and3are not equivalent to the magnetic fieldH0rotated from the [001] to [110] axis. (b) A trigonally distorted VO6ligand field splits a five-fold 3dlevel intoegandt2ghaving lowera1gand upperwith 1.5 electrons. For the2and3sites, the trigonal axis is located at 54° measured from the crystal [001] axis. (c) In a Kondo lattice having localizeda1gand itinerantelectrons with transferst, exchange interactions between the occupied orbitals are composed of the on-site ferromagnetic Hund's couplingJH, the off-diagonal Kondo couplingJKand the off-site antiferromagnetic kinetic exchangeJAF. Figure 1: V pyrochlore lattice and exchange interactions between 3 d orbitals in LiV 2 O 4 . ( a ) Corner-sharing V tetrahedra offer geometric frustration against magnetic ordering. In the cubic lattice with local trigonal distortion, three vanadium sites with a 1g -like orbitals, numbered 1 , 2 and 3 are not equivalent to the magnetic field H 0 rotated from the [001] to [110] axis. ( b ) A trigonally distorted VO 6 ligand field splits a five-fold 3 d level into e g and t 2g having lower a 1g and upper with 1.5 electrons. For the 2 and 3 sites, the trigonal axis is located at 54° measured from the crystal [001] axis. ( c ) In a Kondo lattice having localized a 1g and itinerant electrons with transfers t , exchange interactions between the occupied orbitals are composed of the on-site ferromagnetic Hund's coupling J H , the off-diagonal Kondo coupling J K and the off-site antiferromagnetic kinetic exchange J AF . Full size image Experimentally, the interpretations have been unclear for HQs in LiV 2 O 4 . Charge-sensitive probes such as resistivity [2] , photoemission [13] and optical [14] measurements showed crossover from a high-temperature incoherent metal to a low-temperature Fermi liquid across the characteristic temperature T *~ 20–30 K. In contrast, spin-sensitive probes including static spin susceptibility [2] , [15] and inelastic neutron scattering [16] measurements imply local moments with antiferromagnetic correlations at low temperatures. Furthermore, anomalous temperature T dependences on the specific heat C / T and the Hall coefficient conflict with those expected in a conventional Fermi liquid [2] . Despite the theoretical view of orbital-selective interactions, no experimental effort has been made to detect the orbital degrees of freedom. Here, we address the first experimental approach for microscopic observations of the d HQ via orbital-resolved nuclear magnetic resonance (ORNMR) measurements in LiV 2 O 4 . The previous NMR experiments using closed-shell Li sites [2] , [15] only measured the net spin susceptibility proportional to the bulk value because the hyperfine interactions at the Li site surrounded by 12 vanadium sites average out the anisotropy. Our ORNMR spectroscopic approach using on-site 51 V spins on a high-quality single crystal is sensitive to the orbital-dependent local spin susceptibility, which is beneficial for probing strongly correlated electrons with the orbital degrees of freedom. ORNMR Knight shift In LiV 2 O 4 , the spin susceptibility χ s consists of the a 1g and components: χ s = χ a + χ e (hereafter the superscripts a and e denote a 1g and , respectively). The NMR frequency shift called the Knight shift, ( x , y and z are the principal axes), measures the spin susceptibility via the hyperfine interaction with the hyperfine coupling tensor A i between the nuclear spin I and the paramagnetic spin polarization for the i -th electron under an external magnetic field. Whereas the isotropic shift due to the core polarization is proportional to χ s , the anisotropic part due to the orbital-specific dipole hyperfine interaction [17] is expressed by using the principal z component of the coupling constants, and , where N is Avogadro's number and μ B is the Bohr magneton. In contrast to measures the hyperfine-weighted average of the orbital-dependent spin susceptibility. In the ionic limit, and are given by a quadratic combination of the angular momentum (see Methods ) with the reversed sign and the same amplitude, (ref. 17 ). Hence, we can distinguish which orbital dominates the spin susceptibility from the sign of and obtain the orbital occupation from the amplitude. Namely, should be positive (negative) for χ a > χ e ( χ a < χ e ). The 51 V Knight shift tensors of LiV 2 O 4 are determined from the angle dependence of K for 2–300 K, as shown in Fig. 2 . The 51 V NMR spectra were detectable only at specific angles, where the nuclear quadrupole interaction almost vanishes, because the nuclear spin-spin relaxation times at other angles are too fast. The obtained K traces three cosine curves of equation (2) in the Methods, which satisfies the cubic Fd 3 m lattice. The principal z axis of K at ±54° for the two V sites indicates the 3 d orbital symmetry governed by the trigonal VO 6 crystal field ( Fig. 1b ). At 300 and 2 K, the relationship shows the a 1g -dominant spin susceptibility ( χ a > χ e ). The result is consistent with the localized nature of the a 1g orbital, as theoretically suggested [4] , [5] , [6] , [10] . 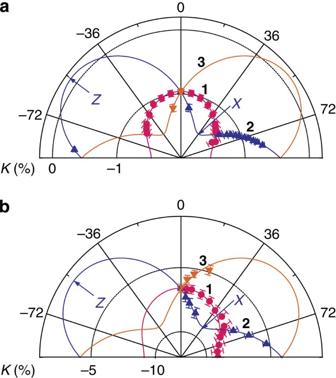Figure 2: Angle dependence of the51V Knight shiftKof LiV2O4. The Knight shiftKmeasured at (a) 300 K and (b) 2 K is plotted against the magnetic field direction measured from the [001] axis to the orthogonal [110] axis. Error bars are defined by a s.d. of the Lorentzian fit of the NMR spectra. Red, blue and orange lines and symbols correspond toKdata from the vanadium sites1,2and3, respectively. The principalZandXaxes ofKfor2and3are, respectively, located at ±54° and ±36° measured from [001]. Figure 2: Angle dependence of the 51 V Knight shift K of LiV 2 O 4 . The Knight shift K measured at ( a ) 300 K and ( b ) 2 K is plotted against the magnetic field direction measured from the [001] axis to the orthogonal [110] axis. Error bars are defined by a s.d. of the Lorentzian fit of the NMR spectra. Red, blue and orange lines and symbols correspond to K data from the vanadium sites 1 , 2 and 3 , respectively. The principal Z and X axes of K for 2 and 3 are, respectively, located at ±54° and ±36° measured from [001]. Full size image Temperature dependence of orbital occupations To address HQ formation, we measured the thermal variations of the 51 V Knight shifts and in comparison with the 7 Li Knight shift and the bulk spin susceptibility χ ( Fig. 3a ). Good linearity was observed between these Knight shifts and χ ( Supplementary Fig. S1 ). All of data show a Curie–Weiss-like increase at high temperatures, followed by a broad maximum at approximately 20 K. The results agree with the spin susceptibility for high-quality crystals, free from a Curie-tail increase at low temperatures [2] , [3] . The on-site 51 V Knight shift probes the spin susceptibility with greater sensitivity than the off-site 7 Li one and shows a smooth decrease below T * . Below 5 K, K s becomes nearly T independent, as observed in the Fermi liquid. 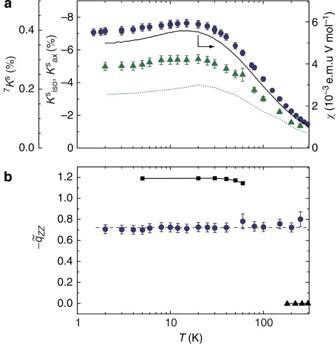Figure 3: Temperature dependence of spin and orbital polarizations in LiV2O4. (a) Local spin susceptibilities probed by51V isotropic shift(circles with error bars), axially anisotropic shift(triangles with error bars) and7Li Knight shift(green dotted line), where error bars are defined by the s.d. The right-hand axis shows the bulk susceptibilityχ(solid curve). A constantK0=0.4% obtained from theK–χplot (Supplementary Fig. S1) is subtracted fromK. (b) The effective 3dorbital polarization(blue circle with error bars) in comparison with the fullya1gpolarized valuein Lu2V2O7(black square)18, and the fully unpolarized valuein a weakly correlated metal V2O3(black circle) (Y.S., M.I., & Y. Ueda, personal communication).is obtained fromdivided byto cancel the spin polarization. Figure 3: Temperature dependence of spin and orbital polarizations in LiV 2 O 4 . ( a ) Local spin susceptibilities probed by 51 V isotropic shift (circles with error bars), axially anisotropic shift (triangles with error bars) and 7 Li Knight shift (green dotted line), where error bars are defined by the s.d. The right-hand axis shows the bulk susceptibility χ (solid curve). A constant K 0 =0.4% obtained from the K – χ plot ( Supplementary Fig. S1 ) is subtracted from K . ( b ) The effective 3 d orbital polarization (blue circle with error bars) in comparison with the fully a 1g polarized value in Lu 2 V 2 O 7 (black square) [18] , and the fully unpolarized value in a weakly correlated metal V 2 O 3 (black circle) (Y.S., M.I., & Y. Ueda, personal communication). is obtained from divided by to cancel the spin polarization. Full size image When a 1g local moments becomes Fermi liquid with HQ via a 1g - hybridization or intersite Kondo coupling below T * , χ a is expected to decrease significantly, whereas χ e is less sensitive. It could lead a decrease of from equation (1). To inspect this property, we plot against T in Fig. 3b . We find no appreciable change in for 2–300 K. This lack of change signifies that the localized character of the a 1g orbital persists to the Fermi liquid state across T * . Although of the f -electron system has not been reported, the non-linear relationship in the K – χ plot may be a manifestation of Kondo coupling in the Ce- and U-based compounds [20] , [21] , [22] . reflects the 3 d orbital polarization when χ a and χ e scale to electron occupations. From we can evaluate the mixing ratio of the a 1g and orbitals in LiV 2 O 4 . The singly occupied a 1g orbital has , as observed in the insulating pyrochlore material Lu 2 V 2 O 7 (ref. 18 ). In contrast, vanishes for equivalent mixing of a 1g and , as observed in a less correlated metal V 2 O 3 ( Fig. 3b ). The observed intermediate in LiV 2 O 4 manifests a significant contribution to the spin susceptibility in throughout the temperature range. Namely, the spin must be polarized via Hund's rule coupling to the localized a 1g spins under the magnetic field, although the itinerancy of is much better than that of a 1g . The occupation ratio is evaluated as (see Methods ), corresponding to the electron numbers of and for 3 d 1.5 . The half-filling a 1g occupation is distinct from that expected in the tight-binding calculation without electron correlations, where (ref. 12 ). However, it is compatible with the strongly localized a 1g picture owing to the strong renormalization into the Mott insulating state [5] , [9] , [10] and provides microscopic evidence for orbital-dependent localization, which is robust across T * . Dynamical spin susceptibility of the orbital-selective spin liquid Another interesting issue is the dynamical part probed by the nuclear spin-lattice relaxation rate . is generally given by (ref. 19 ), where is the wave vector q component of the hyperfine coupling constant normal to the quantization axis, and is the transverse dynamical spin susceptibility at the NMR frequency ω . In a cubic lattice, and are isotropic for the 51 V and 7 Li sites. ( T 1 T ) −1 measured for 51 V and 7 Li ( Fig. 4a ) follows the linear relationship , where the linear coefficient C =1.0×10 3 is close to the square ratio of the hyperfine coupling, and C 0 =64 s −1 K arises from the T -invariant orbital component. The scaling relation indicates that the Li sites probe spin fluctuations via the net transferred hyperfine interaction and allows us to evaluate unobservable at low temperatures from . 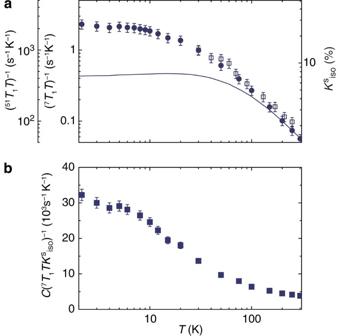Figure 4: The dynamical spin susceptibility compared to a static one in LiV2O4. (a) The temperature dependence of the nuclear spin-lattice relaxation rate divided by temperature, obtained for7Li (solid circle with error bars) and51V (open square with error bars) NMR (left axes) and the isotropic51V Knight shift(solid line, right axis) in LiV2O4, where error bars are defined by the s.d. (b)(solid square with error bars) divided by, whereis equivalent to the spin part of. Figure 4: The dynamical spin susceptibility compared to a static one in LiV 2 O 4 . ( a ) The temperature dependence of the nuclear spin-lattice relaxation rate divided by temperature , obtained for 7 Li (solid circle with error bars) and 51 V (open square with error bars) NMR (left axes) and the isotropic 51 V Knight shift (solid line, right axis) in LiV 2 O 4 , where error bars are defined by the s.d. ( b ) (solid square with error bars) divided by , where is equivalent to the spin part of . Full size image In the present case, is governed by paramagnetic fluctuations of local moments at high temperatures. Above 150 K, the scaling behaviour between and is indeed observed = constant in Fig. 4b ). Below 150 K, a progressive increase indicates antiferromagnetic correlation, consistent with the growth of χ ( q , ω ) at a finite q (=0.64 Å −1 ) in the inelastic neutron scattering measurements below 80 K (ref. 16 ). Therefore, the suppression of χ s at low temperatures likely comes from the short-range antiferromagnetic correlation with the exchange interaction J AF ~150 K. Nevertheless, no long-range magnetic ordering occurs down to 1.5 K, the energy scale of ~ J AF /100. It suggests that the frustrated a 1g spins form in a quantum liquid at low temperatures with low-lying excitations. Our results provide significant insights into the formation of 3 d HQ. As observed in the T -independent , the a 1g spins likely remain incoherent, even entering into a coherent 'Fermi liquid' state, and couple ferromagnetically to spins. No indication of Kondo coupling was observed down to low temperatures despite the large antiferromagnetic fluctuations. The remaining local moments can be highly frustrated and carry large residual entropy [6] , [7] , [8] . The itinerant electrons interact with the underlying spin liquid via the Hund's rule coupling. Thus, the 3 d HQ behaviour in LiV 2 O 4 could be mapped on the frustrated ferromagnetic Kondo lattice. In the absence of antiferromagnetic Kondo coupling, the HQ formation has not been established theoretically. In a Hubbard model calculation, the Kondo-like coherence peak appears on the boundary of the orbital-selective Mott transition for the a 1g part [10] . Even in such a case, χ a may vary across T * , while χ e is invariant. Our results suggest that, if the Kondo-like peak appears, a large fraction of the incoherent spins still remains and carries entropy. Such fractionalization of the nearly localized electron might be common to strongly correlated electron systems [23] , where localized and itinerant characters coexist. Furthermore, the chirality degrees of freedom might provide appreciable entropy in the pyrochlore lattice [24] and contribute to the anomalous Hall effect [3] . The ORNMR technique offers new holographic experiments that could give microscopic insights into strongly correlated electrons. Various orbital-resolved tools, such as X-ray absorption and photoemission spectroscopy, have been recently developed. The Knight shift measurement has a unique advantage in detecting the orbital-dependent local spin susceptibility via the magnetic hyperfine interactions between d spins and on-site nuclear spins. The method has not been achieved in rare-earth heavy fermion compounds because of the difficulty in detecting NMR signals for the on-site nuclear spins [20] . Additional technical improvements in the NMR measurements may reveal the hidden orbital-selective Mott transition in transition metal oxides, such as ruthenates, pnictides and manganites. NMR measurements The ORNMR experiments were performed on a single crystal of LiV 2 O 4 synthesized by the self-flux method [25] . The crystal with the octahedral shape was placed on a two-axis goniometer and rotated under a fixed magnetic field H 0 =9.402 and 8.490 T. The NMR spectra were obtained from spin-echo signals after two π /2 pulses separated by a time τ . The 51 V NMR measurements were made only for powder samples above 50 K (ref. 15 ) likely due to the fast spin-echo decay time T 2 at low temperatures. To overcome this problem, we used a short τ =3–10 μs and a magnetic field precisely (<0.1°) aligned to the crystal axis equivalent to the magic angle of the nuclear quadrupole interaction. Otherwise, the NMR signals were depressed owing to the fast T 2 . The angular dependence of the 51 V Knight shift K(θ ) with the local trigonal symmetry is fitted into the general formula [26] for the V1 site and for the V2 or V3 site related by a mirror symmetry, where Magnetic hyperfine interactions Magnetic hyperfine interactions in 3 d systems are generally given by [17] where l i , s i and I denote operators of orbital and spin of the i -th electron and the nuclear spin, respectively, the coefficient using the Bohr magneton μ B , the nuclear gyromagnetic ratio γ n , the Plank's constant and a radial expectation value r −3 . The first term represents the orbital contribution that quenches in crystals but partly revives via the Van–Vleck process under the magnetic field. The second term arises from a Fermi contact interaction due to the core polarization of inner s spins, giving the isotropic hyperfine coupling constant (κ~0.5 for vanadates [18] , where κ is a dimensionless parameter). The third term denotes anisotropic dipole interactions determined by 3 d orbital occupations, where the principal components are expressed as by using the equivalent operator of 3 d angular momentum, with the spin-orbit coupling parameter λ and the second-order matrix elements between the ground and excited states, . In the LS -coupling, the sum of the terms for several electrons can be replaced by where L and S are total orbital and spin, respectively, and . Analysis of the 51 V Knight shift The experimental observable is the Knight shift tensor K =( K x , K y , K z ) defined as the resonance frequency shift due to the hyperfine interaction of equation (4). The spin component K s is obtained by subtracting the small orbital component K 0 including the chemical shift and the Van–Vleck shift from the K – χ plot in Supplementary Figure S1 . For a paramagnetic system, s i in equation (4) is replaced by the effective electron spin polarization proportional to spin susceptibility χ s . In a multi-orbital system, χ s is composed of orbital-dependent spin susceptibilities. Then K s is expressed by the sum of hyperfine fields from 3 d spins. Whereas the isotropic part of K s , , is given by the anisotropic part, , is expressed as the arithmetic average of the orbital-dependent spin susceptibility weighted by the principal z component of the hyperfine coupling tensor, as shown inequation (1). In LiV 2 O 4 , with a local trigonal distortion, 1.5 electrons are filled in two orbitals, a 1g and , whose q αβ are equivalent to those of and , respectively, taking the principal axes along the trigonal axis: q xx = q yy =1, q zz =−2 for ( a 1g ) 1 , while the values are numerically the same but reversed in sign for . q αα vanishes when the two orbitals are equally occupied. Using the relation is expressed as The good linearity in K – χ plots indicates , where f is the fraction of χ a in χ s . Then can be further reduced to for the negligible as expected from the small K 0 . To experimentally obtain the effective orbital polarization , we take a ratio of Equations (7) and (9)) and cancel out the numerical constants and χ s . Namely, Here for a fully a 1g polarized case ( f =1), close to the experimentally obtained in LuV 2 O 7 (ref. 18 ). From the experimental result in LiV 2 O 4 , we obtained f ~0.8, corresponding to the occupation ratio and hence n ~1 for a 1g and n ~0.25 for . Electric hyperfine interactions The electrostatic hyperfine interaction can be a direct probe for 3 d orbital order. In the presence of the anisotropic electric field gradient around the nuclear spin, the 51 V NMR spectrum is split into seven lines for I =7/2. The NMR spectrum becomes sharpest at [001], identifying the magic angle where the nuclear quadrupole splitting frequency δ v vanishes. Then δ v should have a maximum at θ 0 =54.7° satisfying δ v~ ( 3 cos 2 θ 0 −1)=0, which is exactly equivalent to the local trigonal symmetry. We observed a quadrupole splitting frequency δ v x =90 kHz in the 51 V NMR spectra at H 0 ||[110], by using a very short pulse interval time τ =3 μs. From the lattice symmetry, we can obtain . We confirmed that δ v x was independent of temperature down to 2 K and hence the orbital occupation was invariant across T * . How to cite this article: Shimizu Y. et al . An orbital-selective spin liquid in a frustrated heavy fermion spinel LiV 2 O 4 . Nat. Commun. 3:981 doi: 10.1038/ncomms1979 (2012).